Population structure determines functional differences among species and ecosystem processes Linking the structure of communities to ecosystem functioning has been a perennial challenge in ecology. Studies on ecosystem function are traditionally focused on changes in species composition. However, this species-centric approach neglects the often dramatic changes in the ecology of organisms during their development, thereby limiting our ability to link the structure of populations and communities to the functioning of natural ecosystems. Here we experimentally demonstrate that the impact of organisms on community structure and ecosystem processes often differ more among developmental stages within a species than between species, contrary to current assumptions. Importantly, we show that functional differences between species vary depending on the specific demographic structure of predators. One important implication is that changes in the demography of populations can strongly alter the functional composition of communities and change ecosystem processes long before any species are extirpated from communities. Natural communities are increasingly altered by anthropogenic factors [1] . Unfortunately, the ways ecosystems respond to these community changes often cannot be predicted by classical theory [2] . For instance, although size-selective harvesting of predatory fishes in the Atlantic has not changed their total biomass or diversity for decades, it has dramatically altered community structure and many ecosystem properties [3] . This suggests that current approaches miss important information necessary to predict how changes in the structure of communities will alter the functioning of natural ecosystems. Part of the problem may arise from the coarse resolution of community structure that stems from current species-centric approaches. When facing complex systems like natural communities, the challenge is to identify the scale with which we need to resolve the system to make accurate predictions. Mounting evidence indicates that the ecological differences among organisms in the community (that is, functional diversity) are more important than taxonomic diversity to link community structure and ecosystem functioning [4] , [5] , [6] , [7] , [8] , [9] . Functional diversity, however, is still estimated based on the average traits of a species. A drawback of this species-centric approach is the assumption that the functional role of a species is fixed within a community [4] , [5] , [6] , [7] , [10] , which also implies that functional differences within species are negligible compared with differences among species. This, however, ignores the potential importance of ecological variation among individuals within a species [2] , [11] , [12] , thereby precluding our ability to link changes in population and community structure to ecosystem functioning [13] . By far, the largest source of this intraspecific variation stems from differences in body size and developmental stage [14] , [15] , [16] , [17] . Indeed, ecological differences (for example, diet, habitat use) among stages within species can rival or even exceed differences between species [18] , [19] , [20] . Given such differences among stages, the demographic structure of populations should strongly determine the functional roles of species, thereby influencing ecosystem functioning [21] . Yet, there is considerable debate about whether and how it should be incorporated into current ecological models and conservation efforts [2] , [22] , [23] , [24] , [25] because it is generally assumed that ontogenetic functional variation within species is insignificant compared with functional variation among species at the ecosystem level, although this remains to be tested. To predict how ontogenetic functional diversity influences ecosystem functioning requires an understanding of the magnitude of functional differences among stages, how this compares with functional differences across species, and given that multiple stages commonly co-occur, we need to know whether effects of stages are independent of each other to predict the realized effect of a species on the ecosystem and long-term dynamics. Here we present a novel experiment that manipulates the stage structure of populations for two key predator species in complex experimental communities to examine how changes in the structure of populations are linked to the functional role of a species, functional differences among species and ultimately the structure and processes of complex ecosystems. By measuring nine key ecosystem properties, and identifying, counting, measuring and weighing >35,000 individuals from >65 morphospecies in total, we demonstrate that changes in the demographic (stage) structure of populations scale up to alter the structure and functioning of complex ecosystems, and that functional differences between species are determined by their respective demographic structure. These results indicate that changes in the demography of populations can strongly alter the functional composition of communities and change ecosystem processes long before any species are extirpated from communities. General patterns We found striking differences among treatments across all measured ecosystem properties, ranging from community composition ( Fig. 1 ) and biomass of functional groups ( Fig. 2 ) to ecosystem processes ( Fig. 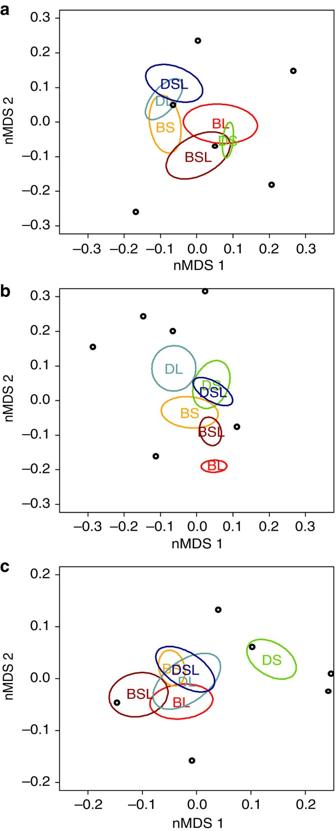Figure 1: Differences in animal community structure. Two non-metric multidimensional scaling (nMDS) axes of (a) proportional abundance and (b) proportional biomass of all animal species, and (c) proportional abundance of different macroinvertebrate size classes for different predator treatments. The ellipse shows the mean (centre of ellipse)±1 s.e.m. of the community structure for each treatment (n=6 per treatment). Letters within an ellipse indicate predator treatments; the first letter indicates the species identity of the predator (D=Dragonfly (Anax), B=Beetle (Cybister), subsequent letters indicate what stages of that predator are present: S=small, L=large and SL=small+large). Black circles indicate individual mesocosm communities in the predator-free control. nMDS two-dimensional stress levels for (a)=0.2, (b)=0.15 and (c)=0.11. SeeTable 1for statistical analysis. 3 ; Table 1 ). Functional differences among populations with different stage structures often rivalled or even exceeded differences among species. Importantly, functional differences among species were typically dependent on the specific stage structure within species ( Table 1 , species × stage). Consequently, the majority of ecosystem properties were jointly determined by the stage and species’ identity of focal predators ( Table 1 ). Figure 1: Differences in animal community structure. Two non-metric multidimensional scaling (nMDS) axes of ( a ) proportional abundance and ( b ) proportional biomass of all animal species, and ( c ) proportional abundance of different macroinvertebrate size classes for different predator treatments. The ellipse shows the mean (centre of ellipse)±1 s.e.m. of the community structure for each treatment ( n =6 per treatment). Letters within an ellipse indicate predator treatments; the first letter indicates the species identity of the predator (D=Dragonfly ( Anax ), B=Beetle ( Cybister ), subsequent letters indicate what stages of that predator are present: S=small, L=large and SL=small+large). Black circles indicate individual mesocosm communities in the predator-free control. nMDS two-dimensional stress levels for ( a )=0.2, ( b )=0.15 and ( c )=0.11. See Table 1 for statistical analysis. 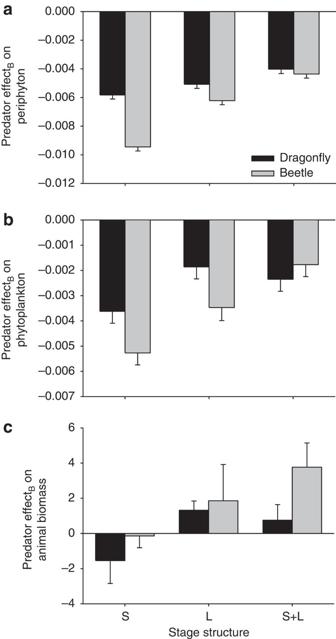Figure 2: Differences in primary producer and animal biomass. Bars indicate treatment means+1 s.e.m., stage structure indicates what stage of a predator species is present: S=small stage, L=large stage, S+L=both stages co-occur. EffectBindicates the standardized per-unit biomass effect (seeSupplementary Methodsfor details) of predators within a given treatment on the respective ecosystem trait relative to the predator-free control. (a) and (b) indicate the proportional change in respective primary producer biomass over the duration of the experiment based on chlorophyll-arelative to the control. (c) Dry biomass of all macroinvertebrates and amphibians at the end of the experiment relative to the control. Each treatment was replicated six times. SeeTable 1for statistical analysis. Full size image Figure 2: Differences in primary producer and animal biomass. Bars indicate treatment means+1 s.e.m., stage structure indicates what stage of a predator species is present: S=small stage, L=large stage, S+L=both stages co-occur. Effect B indicates the standardized per-unit biomass effect (see Supplementary Methods for details) of predators within a given treatment on the respective ecosystem trait relative to the predator-free control. ( a ) and ( b ) indicate the proportional change in respective primary producer biomass over the duration of the experiment based on chlorophyll- a relative to the control. ( c ) Dry biomass of all macroinvertebrates and amphibians at the end of the experiment relative to the control. Each treatment was replicated six times. See Table 1 for statistical analysis. 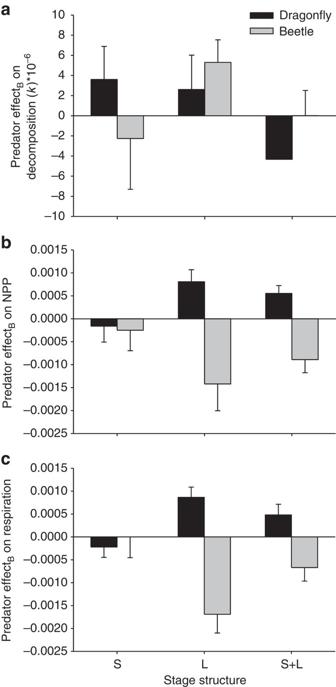Figure 3: Differences in ecosystem processes. Bars indicate treatment means+1 s.e.m., size structure indicates what stage of a predator species is present (seeFig. 2). EffectBindicates the standardized per-unit biomass effect (seeSupplementary Methodsfor details) of predators within a given treatment on the respective ecosystem trait relative to the predator-free control. (a) Decomposition constant (k). (b,c) proportional change in net primary productivity (NPP) and R based on diurnal cycles of dissolved oxygen over the duration of the experiment. Each treatment was replicated six times. SeeTable 1for statistical analysis. Full size image Figure 3: Differences in ecosystem processes. Bars indicate treatment means+1 s.e.m., size structure indicates what stage of a predator species is present (see Fig. 2 ). Effect B indicates the standardized per-unit biomass effect (see Supplementary Methods for details) of predators within a given treatment on the respective ecosystem trait relative to the predator-free control. ( a ) Decomposition constant ( k ). ( b , c ) proportional change in net primary productivity (NPP) and R based on diurnal cycles of dissolved oxygen over the duration of the experiment. Each treatment was replicated six times. See Table 1 for statistical analysis. Full size image Table 1 Effects of species identity and stage structure on ecosystem properties. Full size table Effects on community structure The impact of a predator on community composition was contingent on its stage and species identity regardless of whether community structure was analysed based on biomass or density indices ( Fig. 1 ; Table 1 ). This interaction was caused by several factors. First, the magnitude of stage-specific differences in community composition varied between species (for example, difference in L versus S for dragonfly versus beetle, Fig. 1a ). Second, the difference in community composition among treatments with different predator species was stage specific ( Fig. 1a ). As a consequence, communities could differ more among treatments that received different stages of the same species than treatments with different species ( Fig. 1 ). For instance, communities with large and small dragonfly predators differed much more from each other (based on density indices) than from communities with predatory beetle stages ( Fig. 1a ). In addition, differences among species did not consistently scale with size. For instance, communities with large dragonflies were more similar (based on biomass indices) to communities with small beetles compared with communities with large beetles ( Fig. 1b ), indicating that the size of individuals cannot be used as a surrogate for species either. Community composition was analysed based on the relative abundance/biomass of species within a community, and therefore was corrected for any natural differences in total biomass or density across predator treatments (which was analysed separately, Supplementary Methods ). Consequently, the observed differences in community structure represent true changes in species composition, indicating that stages and species interacted (directly or indirectly) with different components of the food web. Such qualitative differences would not be expected if stages share species interactions and if foraging rates simply scale with differences in predator biomass or size (stage). Interestingly, these differences in species composition across treatments were not reflected in the size structure of the community itself. That is, the relative abundance of different-sized individuals in a community remained comparable across treatments ( Table 1 ; Fig. 1c ). This suggests that change in species composition did not merely result from smaller predator stages consuming more small prey than large predator stages [26] . Given that differences in food web structure were significantly correlated with changes in all ecosystem processes ( Table 2 ), this indicates that changes in the population stage structure of a keystone species translated into changes in the relative abundance of different functional groups within a community. Table 2 General relationships among ecosystem properties. Full size table Effects on functional groups Besides differences in relative community composition, treatments also differed in total biomass across trophic functional groups even after accounting for potential differences in predator biomass across treatments. The per-unit biomass effect of predators on periphyton (benthic algae) and phytoplankton (pelagic algae) biomass was driven by the interaction of species identity and stage structure of populations: although beetles generally had a stronger per-unit biomass effect than dragonflies, the differences were stage specific and disappeared when two stages were present together ( Table 1 ; Fig. 2 ). In contrast, final animal biomass was only affected by predator stage regardless of predator identity ( Table 1 ; Fig. 2 ). Interestingly, small predator stages had a stronger per-unit biomass effect ( Fig. 2 ), and generally reduced total primary producer and animal biomass in mesocosms more than large stages ( Supplementary Fig. S1 ). This occurred despite total biomass of keystone predators in treatments with large predators being similar or slightly higher ( Supplementary Methods ). However, the differences in animal and phytoplankton biomass were significantly correlated with differences in species composition ( Table 2 ), indicating that predator-mediated changes in functional composition of communities were primarily responsible for the observed differences among predator stages. Effects on ecosystem rates Ultimately, stage-specific differences in trophic cascades among keystone predators also resulted in differences in all measured ecosystem processes. Total decomposition rates were only different among mesocosms with different predator stages, regardless of their species identity ( Supplementary Table S1 ; Supplementary Fig. S2 ). However, there was no significant difference in per-unit biomass effect among predator treatments, suggesting that this difference was largely driven by differences in predator biomass across stage treatments ( Table 1 ; Fig. 3 ). The change in net primary productivity (NPP) and respiration (R) during the experiment was affected by the interaction of species identity and stage of the predator treatment ( Table 1 ; Supplementary Table S1 ) and closely followed changes in community composition ( Fig. 1 ; Table 2 ). In both predator species, small stages had significantly different per-unit biomass effects on NPP and R rates than treatments with large stages (all P <0.05, post-hoc test; Fig. 3 ). However, relative differences among stage treatments were opposite in beetle versus dragonfly treatments: in dragonfly treatments, small stages had lower effects on R and NPP, whereas the opposite was true for beetle treatments. Furthermore, small stages of both species had similar effects, whereas large stages had different and even opposite effects across species ( Fig. 3 ). Importantly, this implies that whether species were functionally different or redundant [27] changed depending on which stages are compared. This clearly emphasizes the importance of accounting for stage structure within species when making inferences about a species’ functional role and functional differences among species. Non-additive effects of consumer stages Given that multiple stages co-occur in many species, an important unresolved question is whether the combined effects of different stages on the ecosystem can be predicted by their individual effects or whether indirect interactions among co-occurring stages lead to non-additive effects within species ( Supplementary Methods ). In general, we detected non-additive effects of stages for both species for three out of the six ecosystem properties ( Supplementary Table S2 ; Supplementary Figs S1 and S2 ). The reduction in phytoplankton and decomposition rates in treatments where both stages co-occurred was generally less than expected based on a null model assuming independent (additive) effects of both stages, whereas periphyton biomass was generally larger than expected by the null models. Although such non-additive effects can arise through a range of complex interactions [28] , a more detailed analysis suggests that they probably result from a combination of consumptive (that is, cannibalism) and behavioural mediated interactions among predator stages ( Supplementary Table S2 ). Importantly, this evidence of non-additive, diversity effects within species indicates that we typically cannot average across stages to predict the impact of a species on the functioning of ecosystems. Studies on the relationship between biodiversity and ecosystem functions traditionally focus on species diversity, and implicitly assume that ecological variation within species has little consequences at the ecosystem scale and is insignificant compared with interspecific differences [29] . Our results revealed functional differences among stages at the ecosystem level that rivalled and frequently exceeded differences among species. Furthermore, functional differences among species were contingent on the specific stage structure of the species. These findings indicate that the functional role of a species in a community is not fixed as commonly assumed [4] , [5] , [6] , [7] , [10] but is instead dynamic and varies with changes in the stage/size structure of populations. Given that the majority of animal and plant species (in terrestrial and aquatic systems) experiences shifts in ecological interactions during their ontogeny [2] , [16] , [30] , [31] , our findings likely apply to a broad range of species and systems. Importantly, this implies that changes in the population structure of species can alter the functional composition of communities and lead to concordant changes in ecosystem functioning long before any species are extirpated. This prediction is consistent with observational data on whole ecosystems, where long-term changes in the size/stage structure of predatory fish were correlated with relative changes in the biomasses of lower trophic levels, even when the total biomass of predatory fish remained unchanged [3] , [32] . It also suggests that natural ecosystems are much more sensitive to human disturbances (for example, size-selective harvesting) than previously thought and emphasizes the importance of the demographic structure of populations for conserving ecosystem processes. Identifying functional differences among demographic stages within species is challenging because it requires experiments that are short enough to avoid major stage transitions yet long enough to determine effects on ecosystem processes. Consequently, the duration of this experiment had to be shorter than the generation time of the focal species. However, this is a common scenario in studies on biodiversity and ecosystem function when analysing dynamics across trophic levels, which often vary in generation times, and it does not limit the relevance and importance of the results for predicting the long-term effects on the ecosystem. The stable stage structure of populations is dynamic and varies with natural environmental changes (in space and time) [24] , [33] , [34] . In addition, anthropogenic disturbances, such as size-selective harvesting, habitat fragmentation, invasive species and climate change, have already led to long-term changes in the stage and size structure of many animal and plant species worldwide [3] , [24] , [32] , [35] . Our results indicate that to understand how a species influences long-term dynamics of communities and ecosystems, we need to know how individual stages contribute to the functional role of a species in an ecosystem, and whether there are indirect interactions among stages leading to non-additive (non-independent) effects. In our system, we found dramatic differences in the functional role among stages in both species. In addition, we found that the combined effects of stages are often not independent (that is, not additive), largely because of cannibalistic interactions but also because of other potential non-consumptive indirect interactions. Together, this indicates that any short- or long-term changes in the population stage structure of species will also result in short- and/or long-term changes in ecosystem properties in our and other systems. One of the central challenges in biodiversity research is to identify the appropriate scale at which to resolve communities [2] , [29] . Classical approaches have typically focused on species and estimated functional differences among species based on the average traits of species. Although this work has greatly improved our understanding of the relationship between biodiversity and ecosystems functioning [36] , this approach implicitly assumes that the functional roles of species and thus functional differences among species are fixed traits within a community. Our results are in sharp contrast to this assumption by demonstrating that functional role within and functional differences among species changed during the ontogeny. In some instances, small stages of both predator species had similar effects and large stages differed dramatically (for example, had opposite effects relative to the control), whereas for others small stages were more dissimilar than large stages (for example, Figs 1 and 3 ). This ontogenetic change in species-specific differences could stem from a number of factors that differ among both species, including morphology, behaviour and how gape limitation scales with size ( Supplementary Methods ). There is also no reason to expect that differences among species remain constant over ontogeny. For instance, dragonfly larvae in our system switch in their microhabitat use (from vegetation to leaf litter) during ontogeny [21] , although we did not find a clear indication that this also occurs for beetle larvae. Such differential shifts in microhabitat use could explain why functional differences between species changed during ontogeny. However, predicting the exact underlying mechanisms is challenging because of the complexity (that is, >65 morphospecies) of the system. However, regardless of the exact mechanisms, our results indicate that functional differences among species did not simply scale linearly with size, indicating that we cannot average across stages to estimate functional differences among species. The ontogenetic shifts in functional differences among species highlight a new problem for biodiversity studies: how can we predict ontogenetic shifts in the functional differences among species? Our results clearly indicate that we cannot simply use size (or biomass) as a surrogate for species to predict the functional role of individuals in complex communities. However, there is no a priori reason to assume that functional differences within or among species would scale with size. The impact of individuals on the ecosystem depends on how it alters the functional composition of the community, that is, its direct and indirect interactions. Although interaction strength typically scales with consumer and resource size ratios, the presence/absence of ecological interactions also change with size during ontogeny. In complex communities, such ontogenetic niche shifts can quickly deteriorate the ability of size-differences to explain the impact of individuals on communities and ecosystem processes. Indeed, we found that stages interacted (directly and indirectly) with different components of the food web, indicating ontogenetic niche shifts in ecological interactions that lead to concurrent changes in ecosystem processes. Importantly, the changes in community structure could not be explained by simple shifts in the size structure of the community. This indicates that shifts in ecological interactions did not follow simple size-scaling feeding relationships but instead indicates ontogenetic shifts in behaviour and/or microhabitat use. Such ontogenetic shifts have been recorded in a large variety of vertebrate and invertebrate taxa [16] , [24] . However, although individuals within species clearly can change dramatically in their ecology during ontogeny [16] , [17] , [24] , these changes are still constrained by the basic traits (for example, morphology) of the species itself. For instance, although small stages of both species should be more similar in the size range of prey they consume compared with large stages of both species, what individuals eat will depend on a variety of factors, such as their microhabitat they use, feeding mode and behaviour, all of which will be constrained by their morphologies. As a consequence, similar-sized individuals from different species could have very different effects on community structure as was the case in our study. Thus, future studies that identify how ontogenetic niche shifts in species interactions are constrained by species traits are needed to develop a new general framework that links functional variation within and between species to predict the relationship between community structure and ecosystem processes. Experimental design Larvae of the dragonfly Anax junius and the diving beetle Cybister fimbriolatus were collected from two local ponds in eastern Texas, and stage-specific densities represent natural densities. Although both species are known to be important apex predators (in their final stage) structuring fishless pond communities, they differ in many morphological and behavioural traits and how their morphology changes during development (see Supplementary Methods ). Both species increase by more than 15-fold in length (mass) during their development, and the population structure of both species varies considerably across seasons and populations. Identifying functional differences among very different-sized predators is challenging because individuals differ substantially in their biomass. In traditional designs, predator densities or biomass are often standardized. However, when predators differ substantially in size, such substitutive designs lead to dramatic differences in either biomass or density, and conclusions about identity effects are likely to be confounded by these differences [37] , [38] . Moreover, neither density nor total biomass are ever constant across stage classes within our study species [39] , and keeping total biomass constant would lead to unrealistically high densities of small stages and experimental artifacts. Consequently, in systems where the effects of individuals on the ecosystem are largely driven by body size, there is a high risk of misinterpreting results when using traditional substitutive designs [37] , [40] . Therefore, we refrained from keeping initial biomass or density constant and followed previous suggestions and designs that recommend using natural size–abundance relationships [21] , [37] , [38] , [40] . This approach allowed us to estimate the actual impact of each size class in natural populations and the relative impact of each size class by separating quantitative differences from qualitative differences among size classes. The experiment consisted of seven treatments, each replicated six times ( N =42 ponds) that manipulated the presence and absence of small (S; initial per capita dry mass ~0.026–0.06 mg) and large (L; initial per capita dry mass~0.6 mg) stages of A. junius and C. fimbriolatus separately, resulting in a 2 (species) × 3 (stage combinations: S, L, S+L) factorial design plus one predator-free control treatment. Mesocosms either received 18 small A. junius or 3 large A. junius or both, or 18 small C. fimbriolatus or 3 large C. fimbriolatus or both, or none of these stages (control). The differences in stage structure (one or two stages present) reflect natural differences among populations (ponds) within a time period or seasonal changes within a population. Size classes were chosen based on the size structure of the natural population and to keep total predator biomass (larvae of A. junius or C. fimbriolatus ) within a size class-treatment constant across species, while reducing the risk of early metamorphosis of the largest size class. Thus, density and per capita biomass of individual stages were similar across species and represented natural size–abundance relationships for each species ( Supplementary Methods ). This design allowed us to determine (i) the individual effect of each stage on the ecosystem, (ii) whether effects of stages within species were independent and (iii) whether functional differences among species changed with changes in stage structure within species. Experimental communities and ecosystem properties Mesocosms were constructed in 1,200-l cattle-watering tanks, filled with leaf litter, macrophytes, well water and nutrients. Complex communities were established using a combination of natural colonization of mesocosms and stocking animals from local pond communities. Community structure was estimated from counting, measuring and weighing over 35,500 individuals from >65 species, and included all invertebrates and vertebrates that emerged during the experiment, estimates from subsamples of zooplankton communities and whole-pond samples of all macroinvertebrates and vertebrates that were destructively collected at the end of the experiment ( Supplementary Table S4 ). We also measured total animal biomass, primary producer biomass of benthic (periphyton) and pelagic (phytoplankton) algae using chlorophyll- a extractions, net primary productivity (NPP), respiration (R), and decomposition rates ( k ). Full description of methods is given in Supplementary Methods . All procedures were in compliance with ethical guidelines for animal use and approved by the Institutional Animal Care and Use Committee (IACUC Protocol no. A09022601). Statistical analyses Community structure was analysed using permutational multivariate statistics based on Bray–Curtis similarity metrics, with relative biomass or density of each species (that is, proportion of total community biomass or density of an experimental pond) as dependent variable. This allowed us to isolate treatment effects on community structure after correcting for potential differences in absolute biomass or density across treatments. All other ecosystem properties were analysed using generalized linear models with appropriate error structure in two ways. First, we analysed treatment effects based on untransformed values for all ecosystem properties. Second, to account for any potential differences in biomass effects among predator treatments, we estimated the per capita biomass effect (=effect B ) for each predator treatment (for details, see Supplementary Methods ). Finally, we tested whether stages had independent (additive) effects when they co-occurred using three different null models that assumed additive, multiplicative or biomass-corrected-independent effects of stages. A detailed description of statistical analysis is available in Supplementary Methods . How to cite this article: Rudolf, V. H. W. Rasmussen, N. L., Population structure determines functional differences among species and ecosystem processes. Nat. Commun. 4:2318 doi: 10.1038/ncomms3318 (2013).